Detection of focal adhesion kinase activation at membrane microdomains by fluorescence resonance energy transfer Proper subcellular localization of focal adhesion kinase (FAK) is crucial for many cellular processes. It remains, however, unclear how FAK activity is regulated at subcellular compartments. To visualize the FAK activity at different membrane microdomains, we develop a fluorescence resonance energy transfer (FRET)-based FAK biosensor, and target it into or outside of detergent-resistant membrane (DRM) regions at the plasma membrane. Here we show that, on cell adhesion to extracellular matrix proteins or stimulation by platelet-derived growth factor (PDGF), the FRET responses of DRM-targeting FAK biosensor are stronger than that at non-DRM regions, suggesting that FAK activation can occur at DRM microdomains. Further experiments reveal that the PDGF-induced FAK activation is mediated and maintained by Src activity, whereas FAK activation on cell adhesion is independent of, and in fact essential for the Src activation. Therefore, FAK is activated at membrane microdomains with distinct activation mechanisms in response to different physiological stimuli. Focal adhesion kinase (FAK) localizes at focal adhesions (FAs) on integrin clustering to regulate cell adhesion, migration and mechanotransduction [1] , [2] , [3] . In addition to its crucial roles in the integrin-mediated signalling cascades, FAK regulates cell migration and proliferation in response to growth factors [4] . Because FAK undergoes the association with membrane signalling proteins, such as integrins and growth factor receptors, it is expected that FAK is regulated and activated at the plasma membrane. The plasma membrane has been proposed to contain microdomains enriched with saturated fatty acids and cholesterol [5] . The physical structure of these microdomains is not fully characterized owing to technical limitations. Because these microdomains are insoluble in nonionic detergents, for example, Triton X-100, they are referred as detergent-resistant membrane (DRM) [5] , [6] . Recent evidence suggests that different microdomains at the plasma membrane function as segregated signalling platforms. For example, the kinetics of Src activation, in response to growth factors and pervanadate, was different in and outside DRM regions [7] . Different regulation of Akt was also observed in different membrane microdomains [8] . However, it remains unclear how FAK activation is regulated at different microdomains at the plasma membrane. In addition, the molecular signalling hierarchy governing FAK activation at these subcellular microdomains remains elusive. The traditional detergent extraction method to study molecular signals at membrane microdomains is based on the detergent-resistant property of DRM fractions. However, protein solubility can be changed during detergent treatment, thus the isolated DRM fractions may not correspond to those microdomains in living cells and indeed may originate from other membrane fractions [6] , [9] . In particular, because these microdomains are structurally dynamic [5] , this traditional method is not sufficient to detect signalling events with high spatiotemporal resolution in live cells. Thus, new methods in visualizing FAK activities at membrane microdomains in live cells are of great interests to elucidate the innate FAK functions at these sub-membrane locations. To visualize subcellular molecular events in live cells, genetically encoded biosensors based on fluorescent proteins (FPs) and fluorescence resonance energy transfer (FRET) have been developed [10] . Recently, two FRET-based FAK reporters have been independently developed to detect the conformational change of FAK [11] , [12] . In both reporters, FRET donor FP was fused at the amino terminus of FAK, and acceptor FP was inserted at the linker region between the FERM and kinase domain of FAK. Despite their similar design strategies, the FRET responses of these two reporters on FAK activation were opposite to each other: increasing in one case [12] while decreasing in the other [11] . These observations suggest a complex and unclear FRET mechanism of these reporters. The inserted FP at the linker regions may also partially expose the kinase domain, causing an elevated enzymatic activity of the reporters comparing with the endogenous FAK [11] . This may introduce another layer of complexity when the reporters are expressed in the host cells, possibly by introducing extra enzymatic activity of FAK [11] . Another system consisting of FRET donor and acceptor FPs separately fused to FAK and a double-SH2 domain, respectively, was developed to report the FAK phosphorylation [11] . However, it is difficult to determine whether the FRET signals in this case are engendered from the binding of the double-SH2 domain to the phosphorylated Tyr397 or other tyrosine sites in FAK. Furthermore, because the acceptor/donor ratio at various subcellular locations is not uniform due to the different expression and localization of donors/acceptors, this approach requires more sophisticated mathematical methods to quantify the signals than a simple donor/acceptor ratio. In this study, we have developed a novel FAK biosensor to specifically detect the autophosphorylation at Tyr397 and its subsequent binding to the SH2 domain of Src, which are the crucial molecular events in FAK activation and thus represent the FAK activity [13] . An improved FRET pair, ECFP and YPet, was also utilized to enhance the sensitivity of the biosensor [14] . To monitor the FAK activities at different microdomains of the plasma membrane, this FAK biosensor was further targeted in and outside of DRM regions through lipid modifications, for example, acylation and prenylation [15] . The results showed that the FAK activity at DRM was significantly higher than at non-DRM regions on either integrin-mediated adhesion or platelet-derived growth factor (PDGF) stimulation. Further results indicate that the PDGF-induced FAK activation at DRM is regulated by Src kinase activity. In contrast, the adhesion-induced FAK activation is upstream to the Src activation. These results suggest that DRM microdomains can serve as subcellular platforms for the proper FAK activation, which is involved in distinct molecular hierarchies in response to different physiological stimulations. Design of FAK FRET biosensor and its characterization in vitro We designed a FRET-based FAK biosensor, with a central piece containing the SH2 domain derived from c-Src, a flexible linker peptide, and a specific substrate sequence from FAK encompassing Tyr397, concatenated between ECFP and YPet ( Fig. 1a ). It is expected that Tyr397 in the substrate peptide can be phosphorylated by FAK ( trans- activation) and subsequently bind to the intramolecular SH2 domain, causing a conformation change and a decrease in FRET ( Fig. 1b ). The purified FAK biosensor showed a strong FRET signal ( Fig. 1c , black line). On incubation with FAK, the ECFP emission of the biosensor increased, while that of YPet decreased ( Fig. 1c , red line), suggesting an increase in the ECFP/YPet ratio and hence a decrease in FRET. The quantified results further revealed that the ECFP/YPet emission ratio of the biosensor had a surprisingly high change around 90% on FAK incubation ( Fig. 1d , black circles). This FRET response was eliminated by a specific FAK inhibitor PF573228 (PF228, 1 μM), or a mutation of Tyr397 to Phe in the substrate peptide (FAK YF mutant) ( Fig. 1d ). These results suggest that the FRET change of the biosensor is due to the phosphorylation of the biosensor specifically by FAK, which was further confirmed by western blot analysis ( Fig. 1e ). Importantly, no FRET change of the biosensor was observed on Src incubation ( Fig. 1d ), which was previously shown to cause significant FRET changes of Src FRET biosensors [14] , [16] . These results suggest that the biosensor reports the FAK activity in vitro , but not that of Src, a kinase well regarded to accompany and coordinate closely with FAK in many cellular events [17] . 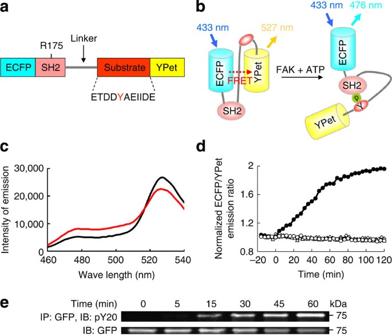Figure 1: The design of the FRET-based FAK biosensor andin vitrocharacterization. (a) The design of FAK biosensor. The FAK biosensor is composed of ECFP, the SH2 domain derived from c-Src, flexible linker, substrate peptide, and YPet. The substrate peptide is derived from FAK containing Tyr397 (indicated as red Y). (b) The principle of the biosensor response. Active FAK can phosphorylate the substrate peptide in the FAK biosensor (indicated as Y), which subsequently binds to the intramolecular SH2 domain to cause a FRET decrease. (c) Emission spectra of the purified FAK biosensor before (black line) and after (red line) the phosphorylation by FAK for 2 h. (d) The time course of the ECFP/YPet emission ratio of FAK biosensor (1 μM) before and after the incubation with FAK (black circles), FAK in the presence of 1 μM PF228 (white diamonds), or Src (white circles). The time course of FRET ratios of FAK YF mutant biosensor (1 μM) was also shown (white triangles). The ECFP/Ypet ratios were normalized against the averaged values before enzyme incubation. (e) The tyrosine phosphorylation level of the FAK biosensor before and after the incubation with FAK. The tyrosine phosphorylation level and total amount of the biosensor, immunoprecipitated from MEF cells, were detected by an anti-phosphotyrosine (pY20) and anti-GFP antibody, respectively. Figure 1: The design of the FRET-based FAK biosensor and in vitro characterization. ( a ) The design of FAK biosensor. The FAK biosensor is composed of ECFP, the SH2 domain derived from c-Src, flexible linker, substrate peptide, and YPet. The substrate peptide is derived from FAK containing Tyr397 (indicated as red Y). ( b ) The principle of the biosensor response. Active FAK can phosphorylate the substrate peptide in the FAK biosensor (indicated as Y), which subsequently binds to the intramolecular SH2 domain to cause a FRET decrease. ( c ) Emission spectra of the purified FAK biosensor before (black line) and after (red line) the phosphorylation by FAK for 2 h. ( d ) The time course of the ECFP/YPet emission ratio of FAK biosensor (1 μM) before and after the incubation with FAK (black circles), FAK in the presence of 1 μM PF228 (white diamonds), or Src (white circles). The time course of FRET ratios of FAK YF mutant biosensor (1 μM) was also shown (white triangles). The ECFP/Ypet ratios were normalized against the averaged values before enzyme incubation. ( e ) The tyrosine phosphorylation level of the FAK biosensor before and after the incubation with FAK. The tyrosine phosphorylation level and total amount of the biosensor, immunoprecipitated from MEF cells, were detected by an anti-phosphotyrosine (pY20) and anti-GFP antibody, respectively. Full size image Characterization of the FAK biosensor in mammalian cells We then examined the FAK biosensor in mammalian cells. The ECFP/YPet emission ratios of the FAK biosensor were significantly higher in mouse embryonic fibroblasts (MEFs) adhered on fibronectin (Fn) than those in suspension ( Fig. 2a ), consistent with the knowledge that the integrin-mediated cell adhesion can induce FAK activation [1] . In contrast, no FRET change was observed in FAK −/− MEFs ( Fig. 2a ), suggesting the specificity of the biosensor in reporting the FAK activity. To further examine its specificity, we introduced the FAK biosensor together with wild-type FAK or its various mutants in FAK −/− MEFs, and measured the FRET levels in these cells adhered on Fn ( Fig. 2b , white bars). The constitutively active FAK (FAK Δ1–375) [18] , and wild-type FAK (FAK WT) caused significantly higher ECFP/YPet emission ratios than the negative mutant of FAK (FAK NT) [18] , kinase-dead FAK (FAK KD), or empty vector. Consistent with the in vitro results ( Fig. 1d ), the expression of wild-type Src (Src WT) caused no significant FRET change of the FAK biosensor in FAK −/− cells. These results suggest that the FAK biosensor can specifically detect the adhesion-induced FAK activation in mammalian cells. The mutation of either the substrate Tyr397 to Phe (YF) or Arg175 to Val (RV) in the SH2 domain of the biosensor eliminated the FRET response of the FAK biosensor in FAK −/− cells expressing the active FAK Δ1–375 ( Fig. 2b , black bars). These results verify our design strategy that the FRET response of the biosensor on FAK activation is due to the intramolecular interaction between the phosphorylated substrate and the SH2 domain. Consistently, strong phosphorylation was observed only in the groups where the wild-type biosensor was expressed together with FAK Δ1–375 or FAK WT ( Fig. 2c ). These results indicate that, in mammalian cells, the substrate tyrosine is specifically phosphorylated by FAK to result in the FRET change of the biosensor. 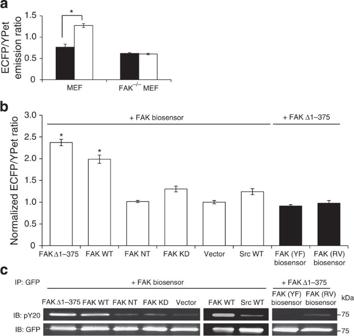Figure 2: The specificity of the FAK biosensor in mammalian cells. (a) The ECFP/YPet emission ratios (mean±s.e.m.) of the FAK biosensor in MEF cells in suspension (n=30) or adhered on Fn(n=10), and in FAK−/−cells in suspension (n=23) or adhered on Fn(n=28). *P=0.001 from student two-tailedt-test. (b) The ECFP/YPet emission ratios of the FAK biosensor (white bars) in FAK−/−MEF cells co-expressing various constructs as indicated: FAK Δ1–375, the constitutively active FAK with the 1–375 amino acids truncated from the full-length FAK (n=18); FAK WT, wild-type FAK (n=13); FAK NT, the negative mutant of FAK containing the N-terminal 1–400 amino acids (n=17); FAK KD, the kinase-dead FAK (n=15); Vector, empty vector pcDNA3 (n=12); Src WT, wild-type Src) (n=24), and the ECFP/YPet emission ratios of the FAK mutant biosensor (black bars), YF (substrate tyrosine mutated,n=11) and RV (SH2 domain disrupted,n=21), in FAK−/−MEF cells coexpressing FAK Δ1–375. All values are shown as mean±s.e.m. and * represents the significant difference from other groups based on the multiple comparison test in Matlab. (c) The tyrosine phosphorylation and expression levels of the FAK biosensor or mutant biosensors (YF and RV) in the groups as described in (b). The tyrosine phosphorylation level and total amount of the biosensor, immunoprecipitated by an anti-GFP antibody from MEF cells, were detected by an anti-phosphotyrosine (pY20) and anti-GFP antibody, respectively. Figure 2: The specificity of the FAK biosensor in mammalian cells. ( a ) The ECFP/YPet emission ratios (mean±s.e.m.) of the FAK biosensor in MEF cells in suspension ( n =30) or adhered on F n ( n =10), and in FAK −/− cells in suspension ( n =23) or adhered on F n ( n =28). * P =0.001 from student two-tailed t -test. ( b ) The ECFP/YPet emission ratios of the FAK biosensor (white bars) in FAK −/− MEF cells co-expressing various constructs as indicated: FAK Δ1–375, the constitutively active FAK with the 1–375 amino acids truncated from the full-length FAK ( n =18); FAK WT, wild-type FAK ( n =13); FAK NT, the negative mutant of FAK containing the N-terminal 1–400 amino acids ( n =17); FAK KD, the kinase-dead FAK ( n =15); Vector, empty vector pcDNA3 ( n =12); Src WT, wild-type Src) ( n =24), and the ECFP/YPet emission ratios of the FAK mutant biosensor (black bars), YF (substrate tyrosine mutated, n =11) and RV (SH2 domain disrupted, n =21), in FAK −/− MEF cells coexpressing FAK Δ1–375. All values are shown as mean±s.e.m. and * represents the significant difference from other groups based on the multiple comparison test in Matlab. ( c ) The tyrosine phosphorylation and expression levels of the FAK biosensor or mutant biosensors (YF and RV) in the groups as described in ( b ). The tyrosine phosphorylation level and total amount of the biosensor, immunoprecipitated by an anti-GFP antibody from MEF cells, were detected by an anti-phosphotyrosine (pY20) and anti-GFP antibody, respectively. Full size image The FAK activity at different microdomains of plasma membrane FAK can be activated at the plasma membrane, which contains different microdomains. Recent evidence suggests that FAK can localize at DRM microdomains [19] , and may regulate the subcellular localization of these membrane microdomains [20] . To observe the FAK activity at DRM regions, Lyn–FAK biosensor was constructed by fusing a DRM-targeting motif containing myristoylation and palmitoylation sites (glycine and cysteine) derived from Lyn, at the N-terminus of the cytosolic FAK (Cyto-FAK) biosensor ( Fig. 3a ) [15] . In parallel, a polybasic-geranylgeranyl motif (cysteine) adapted from K-Ras, was fused at the carboxy terminus of the Cyto-FAK biosensor for the generation of KRas–FAK biosensor that can localize at the general membrane area outside DRM regions ( Fig. 3a ) [15] . When the cysteine in Lyn- and Kras-tags, which is the site for lipid modifications, was mutated to serine, these Lyn and KRas(CS)–FAK biosensors could not correctly localize at the plasma membrane ( Supplementary Fig. S1 ), suggesting that lipid modification is crucial for their subcellular localization at membrane microdomains. The result of sucrose density gradient fractionation further confirmed that Lyn–FAK biosensor was detected in the DRM fraction marked by an endogenous DRM-indicator caveolin-1, whereas KRas–FAK biosensor appeared in the fraction representing the general membrane regions but excluded from DRM ( Fig. 3b ). Similar results have been reported to verify the correct localization of Lyn- and KRas-modified proteins [8] , [15] . Therefore, these results suggest that Lyn- and KRas–FAK biosensors can be successfully targeted into different microdomains of the plasma membrane through different lipid modifications. 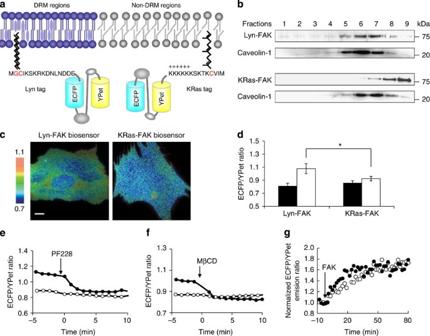Figure 3: The FAK biosensors targeted to the different compartments at plasma membrane. (a) The design of membrane compartment-targeting FAK biosensors. The N-terminal Lyn tag can mediate the acylation of the biosensor to target it into DRM microdomains. The C-terminal KRas tag contains prenylation site and basic residues to target the biosensor to non-DRM regions at plasma membrane. (b) Sucrose gradient fractions of MEF cells expressing Lyn- or KRas–FAK biosensor. The fractions of each biosensor were analysed by western blot with an anti-GFP antibody, and DRM regions were marked by an antibody for caveolin-1. (c) The representative ECFP/YPet ratio images of Lyn–FAK and KRas–FAK biosensors expressed in MEF cells. The colour bar represents the ECFP/YPet ratio values. (Scale bar, 10 μm) (d) The ECFP/YPet emission ratio values (mean±s.e.m.) of Lyn–FAK and KRas–FAK biosensors expressed in the adherent (on Fn, white bars,n=14 for Lyn andn=9 for KRas) and suspended MEF cells (black bars,n=20 for Lyn and n-14 for KRas). *P=0.036 from student two-tailedt-test. (e) The representative time course of the ECFP/YPet emission ratios of Lyn–FAK (black circles,n=5) and KRas–FAK (open circles,n=4) biosensors in response to 1 μM of PF228. (f) The representative time course of the ECFP/YPet emission ratios of Lyn–FAK (black circles,n=5) and KRas–FAK (open circles,n=3) biosensors in response to 5 mM of MβCD. (g)In vitrokinase assays of the Lyn–FAK and KRas–FAK biosensors. The time courses of the normalized ECFP (478 nm)/YPet (526 nm) emission ratio of the purified Lyn–FAK (black circles) and KRas–FAK biosensor (white circles) were shown before and after the incubation with active FAK. The emission ratios were normalized against the averaged signals before the stimulation. Figure 3: The FAK biosensors targeted to the different compartments at plasma membrane. ( a ) The design of membrane compartment-targeting FAK biosensors. The N-terminal Lyn tag can mediate the acylation of the biosensor to target it into DRM microdomains. The C-terminal KRas tag contains prenylation site and basic residues to target the biosensor to non-DRM regions at plasma membrane. ( b ) Sucrose gradient fractions of MEF cells expressing Lyn- or KRas–FAK biosensor. The fractions of each biosensor were analysed by western blot with an anti-GFP antibody, and DRM regions were marked by an antibody for caveolin-1. ( c ) The representative ECFP/YPet ratio images of Lyn–FAK and KRas–FAK biosensors expressed in MEF cells. The colour bar represents the ECFP/YPet ratio values. (Scale bar, 10 μm) ( d ) The ECFP/YPet emission ratio values (mean±s.e.m.) of Lyn–FAK and KRas–FAK biosensors expressed in the adherent (on F n , white bars, n =14 for Lyn and n =9 for KRas) and suspended MEF cells (black bars, n =20 for Lyn and n-14 for KRas). * P =0.036 from student two-tailed t -test. ( e ) The representative time course of the ECFP/YPet emission ratios of Lyn–FAK (black circles, n =5) and KRas–FAK (open circles, n =4) biosensors in response to 1 μM of PF228. ( f ) The representative time course of the ECFP/YPet emission ratios of Lyn–FAK (black circles, n =5) and KRas–FAK (open circles, n =3) biosensors in response to 5 mM of MβCD. ( g ) In vitro kinase assays of the Lyn–FAK and KRas–FAK biosensors. The time courses of the normalized ECFP (478 nm)/YPet (526 nm) emission ratio of the purified Lyn–FAK (black circles) and KRas–FAK biosensor (white circles) were shown before and after the incubation with active FAK. The emission ratios were normalized against the averaged signals before the stimulation. Full size image We next examined the FAK activity at membrane microdomains on MEF adhesion on Fn. Lyn–FAK biosensor tethered at DRM regions showed a significantly higher ECFP/YPet level comparing with KRas–FAK biosensor ( Fig. 3c,d ). The ECFP/YPet ratio of the Lyn–FAK biosensor, but not the KRas–FAK biosensor, decreased from 1.1–0.9 in adherent cells on the incubation of the FAK inhibitor PF228 ( Fig. 3e ). The treatment of methyl-β-cyclodextrin (MβCD), which can extract cholesterol and thus disrupt the microdomain structure, decreased the ECFP/Ypet ratio of Lyn–FAK biosensor, but not KRas–FAK biosensor ( Fig. 3f ). These results suggest that FAK activity is higher inside DRM than non-DRM regions. The minimal response of KRas–FAK biosensor ( Fig. 3c,d ) should be due to the lack of local FAK activity outside DRM regions, but not the steric difficulty of KRas-tagged biosensor in undergoing conformational changes or the activation preference of PDGFR/integrins at DRM microdomains, because Kras–Src biosensor, anchoring outside DRM regions with the same targeting strategy as KRas–FAK biosensor, can be markedly activated on cell adhesion ( Supplementary Fig. S2 ) or PDGF stimulation [7] . In vitro kinase assay further revealed that FAK can cause the similar FRET responses of the purified Lyn– and KRas–FAK biosensors ( Fig. 3g ). Therefore, the different FRET responses of Lyn– and KRas–FAK biosensors in cells are not because of their different membrane-targeting tags but reflecting the differential local FAK activities at membrane microdomains. Although Lyn–FAK biosensor does not contain specific anchoring domain at FA sites, the ECFP/YPet ratios were higher at FAs on adhesion ( Supplementary Fig. S3a ). In fact, the difference of ECFP/YPet ratios of Lyn–FAK biosensor in and outside FAs was significantly higher than that of KRas–FAK biosensor ( Supplementary Fig. S3b ). These results indicate that the FAK activation at FAs can be more correlated with DRM regions and hence more efficiently visualized by Lyn–FAK biosensor. It is also of note that there is a substantial activation of Lyn–FAK biosensor at perinuclear regions ( Supplementary Fig. S3a ). This could be attributed to two potential reasons: the trapped Lyn–FAK biosensor in the recycling pathway including Golgi complex may have higher ECFP/YPet ratios due to the abnormal biosensor conformation/maturation or unusual compartmental environment; or the small FA sites concentrated underneath the perinuclear regions may contain active FAK to phosphorylate Lyn–FAK biosensor anchoring on the plasma membrane within these regions. However, these signals have no obvious contribution to the overall FRET levels as there was no detectable difference when we compared the FRET levels collected from whole-cell body and those from cell periphery (the most peripheral layer if the cell body is divided into five layers, according to the normalized distance to the cell centroid). The PDGF-induced FAK activation at DRM regions We then investigated the FAK activation in and outside DRM regions in response to PDGF stimulation. Lyn–FAK biosensor at DRM regions showed 15–20% increase in ECFP/Ypet ratio within 10 min of PDGF stimulation, whereas KRas–FAK biosensor had only a minimal FRET change (<5%) ( Fig. 4a,b ; Supplementary Movie 1 ). The negative mutant of Lyn–FAK (YF) biosensor also showed a minimal response ( Fig. 4b ), suggesting that the phosphorylation at the designed tyrosine site is responsible for the PDGF-induced FRET change. Biochemical Western blot assay further confirmed that the Lyn–FAK biosensor phosphorylation showed a similar pattern as the Tyr397 phosphorylation of the endogenous FAK ( Fig. 4c ). PF228 reversed the PDGF-induced FRET response of Lyn–FAK biosensor ( Fig. 4d,e ; Supplementary Movie 2 ) without any effect on the PDGFR phosphorylation ( Fig. 4f ), verifying the high specificity of the biosensor in reporting the PDGF-induced FAK activation. The PDGF-induced FRET signal of Lyn–FAK biosensor was also suppressed by MβCD ( Fig. 4d,e ), confirming the localization and functionality of Lyn–FAK biosensor at DRM regions. It is clear that the DRM microdomain structure is critical for the overall FAK activation under different physiological conditions. The PDGF-induced FAK activation occurred predominantly at DRM regions, but not at non-DRM regions ( Fig. 4a,b ) or cytosol ( Supplementary Fig. S4a ). Under adhesion process, FAK activity at DRM regions also has a crucial role in regulating and maintaining the cytosolic FAK activity, because the ECFP/Ypet ratio of cytosolic FAK biosensor was significantly decreased by MβCD ( Supplementary Fig. S4b ). 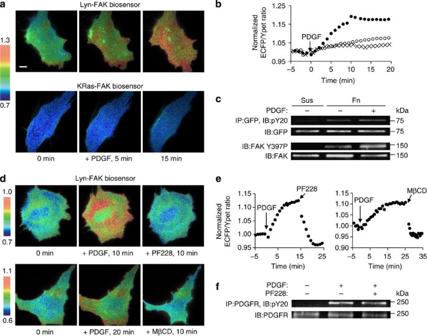Figure 4: The PDGF-induced FAK activation at lipid rafts. (a) The representative ECFP/YPet ratio images of Lyn–FAK and KRas–FAK biosensors on 10 ng ml−1of PDGF stimulation (Scale bar, 10 μm). (b) The representative time courses of the normalized ECFP/YPet emission ratio of Lyn–FAK biosensor (black circles), KRas–FAK biosensor (white circles), and Lyn–FAK (YF) mutant biosensor (x symbol) before and after the PDGF stimulation. To calculate the normalized ECFP/Ypet ratios, we measured the ECFP/Ypet ratios without stimulation and averaged them to obtain a basal level. The ECFP/Ypet ratios at each time point after stimulation was then divided by this basal level to obtain the normalized ECFP/YPet ratio. (c) The phosphorylation and expression levels of Lyn–FAK biosensor and the endogenous FAK Tyr397 from cells in suspension (Sus) or those adhered on fibronectin (Fn) before and after PDGF stimulation. The tyrosine phosphorylation level and total amount of the biosensor, immunoprecipitated by anti-GFP antibody from MEF cells, were detected by an anti-phosphotyrosine (pY20) and anti-GFP antibody, respectively. The phosphorylation and the expression of endogenous FAK were detected by an anti-phosphor-Tyr397 antibody and anti-FAK antibody, respectively. (d,e) The representative ECFP/YPet emission ratio images (d) and normalized time course (e) of Lyn–FAK biosensor in response to PDGF stimulation, with a subsequent treatment of 1 μM PF228 (n=5) or 2.5 mM of MβCD (n=4). (f) PDGF-induced tyrosine phosphorylation level of the PDGF receptor (PDGFR) with and without the pretreatment by 1 μM PF228. The PDGF receptors were immunoprecipitated from MEF cells. Overall tyrosine phosphorylation of PDGFR was detected by immunoblotting with an anti-phosphotyrosine antibody (pY20), and the total amount of PDGFR was measured by the anti-PDGFR antibody. Figure 4: The PDGF-induced FAK activation at lipid rafts. ( a ) The representative ECFP/YPet ratio images of Lyn–FAK and KRas–FAK biosensors on 10 ng ml −1 of PDGF stimulation (Scale bar, 10 μm). ( b ) The representative time courses of the normalized ECFP/YPet emission ratio of Lyn–FAK biosensor (black circles), KRas–FAK biosensor (white circles), and Lyn–FAK (YF) mutant biosensor (x symbol) before and after the PDGF stimulation. To calculate the normalized ECFP/Ypet ratios, we measured the ECFP/Ypet ratios without stimulation and averaged them to obtain a basal level. The ECFP/Ypet ratios at each time point after stimulation was then divided by this basal level to obtain the normalized ECFP/YPet ratio. ( c ) The phosphorylation and expression levels of Lyn–FAK biosensor and the endogenous FAK Tyr397 from cells in suspension (Sus) or those adhered on fibronectin (Fn) before and after PDGF stimulation. The tyrosine phosphorylation level and total amount of the biosensor, immunoprecipitated by anti-GFP antibody from MEF cells, were detected by an anti-phosphotyrosine (pY20) and anti-GFP antibody, respectively. The phosphorylation and the expression of endogenous FAK were detected by an anti-phosphor-Tyr397 antibody and anti-FAK antibody, respectively. ( d , e ) The representative ECFP/YPet emission ratio images ( d ) and normalized time course ( e ) of Lyn–FAK biosensor in response to PDGF stimulation, with a subsequent treatment of 1 μM PF228 ( n =5) or 2.5 mM of MβCD ( n =4). ( f ) PDGF-induced tyrosine phosphorylation level of the PDGF receptor (PDGFR) with and without the pretreatment by 1 μM PF228. The PDGF receptors were immunoprecipitated from MEF cells. Overall tyrosine phosphorylation of PDGFR was detected by immunoblotting with an anti-phosphotyrosine antibody (pY20), and the total amount of PDGFR was measured by the anti-PDGFR antibody. Full size image Src activity is required for the PDGF-induced FAK activation Previous studies showed that, in response to PDGF, FAK can associate with Src (ref. 4 ) and PI3K (ref. 21 ) to regulate downstream signalling cascades and cellular processes. We first investigated the molecular hierarchy regulating FAK and Src activations at DRM regions in response to PDGF. PP1, a Src kinase inhibitor, completely blocked the PDGF-induced FRET response of Lyn–FAK biosensor ( Fig. 5a ; Supplementary Movie 3 ). This PDGF-induced FAK activation was also inhibited in Src/Yes/Fyn triple-knockout (SYF −/− ) MEFs ( Supplementary Fig. S5 ), These results suggest that Src activity mediates the FAK activation in response to PDGF. We then asked whether FAK also regulates Src activation in response to PDGF. We previously developed an improved Src biosensor based on ECFP and YPet [14] . In this study, we targeted this biosensor into DRM regions (Lyn–Src biosensor) to study the molecular interrelation between Src and FAK within these microdomains. 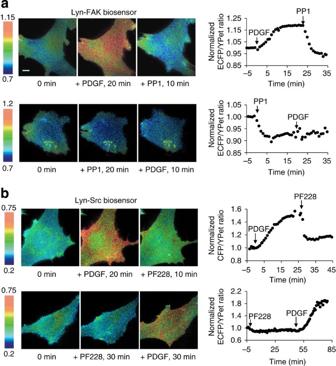Figure 5: Src activity is essential for the FAK activation in response to PDGF stimulation. (a) The representative images and time courses of the normalized ECFP/YPet emission ratio of Lyn–FAK biosensor in response to 10 ng ml−1PDGF in cells subjected to treatments with 10 μM of PP1. Panels show the results of post-PDGF (n=5), and pre-PDGF treatments (n=6), as indicated. (b) The representative images and time courses of the normalized ECFP/YPet emission ratio of Lyn-Src biosensor in response to 10 ng ml−1PDGF in cells subjected to treatments with 1 μM of PF228. Panels show the results of post-PDGF (n=3), and pre-PDGF treatments (n=3), as indicated. The time course emission ratios were normalized against the averaged signals before the stimulation. (Scale bar, 10 μm) As shown in Figure 5b , the PDGF-induced FRET response of Lyn–Src biosensor was only partially reversed by PF228. Furthermore, PF228 did not prevent the PDGF-induced response of Lyn–Src biosensor ( Fig. 5b ), suggesting that FAK activity is not required for the PDGF-induced Src activation. The portion of the Src activity that was sensitive to the FAK inhibitor may be attributed to the adhesion-dependent Src activation, mediated by FAK via its Tyr397 phosphorylation [17] . Figure 5: Src activity is essential for the FAK activation in response to PDGF stimulation. ( a ) The representative images and time courses of the normalized ECFP/YPet emission ratio of Lyn–FAK biosensor in response to 10 ng ml −1 PDGF in cells subjected to treatments with 10 μM of PP1. Panels show the results of post-PDGF ( n =5), and pre-PDGF treatments ( n =6), as indicated. ( b ) The representative images and time courses of the normalized ECFP/YPet emission ratio of Lyn-Src biosensor in response to 10 ng ml −1 PDGF in cells subjected to treatments with 1 μM of PF228. Panels show the results of post-PDGF ( n =3), and pre-PDGF treatments ( n =3), as indicated. The time course emission ratios were normalized against the averaged signals before the stimulation. (Scale bar, 10 μm) Full size image We further examined whether PI3K activity is crucial for the FAK/Src activation in response to PDGF. As an indicator of PI3K activity, we used a GFP-tagged Akt PH domain [22] , which can bind to PIP 3 (a product of PI3K activity) and then translocate to the plasma membrane on PI3K activation [23] , [24] ( Supplementary Fig. S6a ; Supplementary Movie 4 ). A specific PI3K inhibitor LY294002 (LY), which clearly inhibited the PDGF-induced PI3K activation ( Supplementary Fig. S6b ), did not have any effect on the activation of either FAK or Src ( Supplementary Fig. S7a,b ), suggesting PI3K is not essential for the FAK/Src activation in response to PDGF. FAK activity is essential for Src activation on cell adhesion We further explored the molecular relationship between FAK and Src at DRM regions during cell adhesion process. The adhesion-induced FAK activation was not inhibited by PP1 ( Fig. 6a ), but was abolished in SYF −/− cells. The reconstitution of SYF −/− cells with either wild-type Src or kinase-dead Src restored the adhesion-mediated FAK activation ( Fig. 6a ). These results indicate that the Src activity is not required for the FAK activation during adhesion process. Instead, other scaffolding domains of Src, for example, SH2 and SH3 domains, may be important in this case. 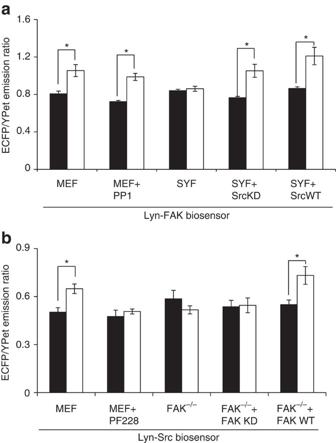Figure 6: FAK acts upstream to Src during the cell-ECM adhesion. The ECFP/YPet emission ratios (mean±s.e.m.) of (a) Lyn–FAK biosensor and (b) Lyn-Src biosensor, in the adherent (on Fn for 1 h, white bars) and suspended cells (black bars). In (a), the groups of cells include MEF, MEF+PP1 (MEFs pre-treated with 10 μM PP1 for 1 h), SYF (SYF−/−cells), SYF+SrcKD (SYF−/−cells reconstituted with the kinase-dead Src), or SYF+SrcWT (SYF−/−cells reconstituted with the wild-type Src). *P=0.002 (MEF group), 0.0001 (MEF+PP1), 0.001 (SYF+SrcKD), and 0.006 (SYF+SrcWT) from student two-tailedt-test. In (b), the groups of cells include MEF, MEF+PF228 (MEFs pre-treated with 1 μM PF228 for 1 h), FAK−/−(FAK knockout MEFs), FAK−/−+FAK KD (FAK−/−cells reconstituted with the kinase-dead FAK), or FAK−/−+FAK WT (FAK−/−cells reconstituted with the wild-type FAK). *P=0.001 (MEF and FAK−/−+FAK WT groups) from student two-tailedt-test. (n=10–30). Figure 6: FAK acts upstream to Src during the cell-ECM adhesion. The ECFP/YPet emission ratios (mean±s.e.m.) of ( a ) Lyn–FAK biosensor and ( b ) Lyn-Src biosensor, in the adherent (on Fn for 1 h, white bars) and suspended cells (black bars). In ( a ), the groups of cells include MEF, MEF+PP1 (MEFs pre-treated with 10 μM PP1 for 1 h), SYF (SYF −/− cells), SYF+SrcKD (SYF −/− cells reconstituted with the kinase-dead Src), or SYF+SrcWT (SYF −/− cells reconstituted with the wild-type Src). * P =0.002 (MEF group), 0.0001 (MEF+PP1), 0.001 (SYF+SrcKD), and 0.006 (SYF+SrcWT) from student two-tailed t -test. In ( b ), the groups of cells include MEF, MEF+PF228 (MEFs pre-treated with 1 μM PF228 for 1 h), FAK −/− (FAK knockout MEFs), FAK −/− +FAK KD (FAK −/− cells reconstituted with the kinase-dead FAK), or FAK −/− +FAK WT (FAK −/− cells reconstituted with the wild-type FAK). * P =0.001 (MEF and FAK −/− +FAK WT groups) from student two-tailed t -test. ( n =10–30). Full size image We next asked whether the FAK activity is required for the adhesion-induced Src activation. As shown in Figure 6b , the inhibition of FAK activity by PF228 completely blocked the adhesion-induced Src activation. This adhesion-induced Src activation is also abolished in FAK −/− fibroblasts, which can be restored only by wild-type FAK, but not kinase-dead FAK ( Fig. 6b ). Therefore, in contrast to the PDGF-induced signalling pathway, the adhesion-mediated FAK activation is required for Src activation. Again, LY did not show any significant inhibitory effect on the adhesion-induced FAK/Src activations ( Supplementary Fig. S7c,d ), suggesting that PI3K activity is not required. FAK serves as a crucial integrator for various signalling networks in cell migration, mechanotransduction and cancer development [25] , [26] . These FAK functions are dependent on its subcellular locations due to different sets and concentrations of molecular intermediates at subcellular regions. For example, FAK promotes the dynamics of FAs [27] , but inhibits that of invadopodia [28] . Therefore, FAK functions and their related molecular hierarchy should be investigated at the subcellular context. Recent evidence suggests that DRM microdomains can guide the subcellular localization and activation of signalling molecules [19] , [20] , [29] . Indeed, whereas PDGF only induced a weak protein phosphorylation outside DRM, a significant increase in protein phosphorylation can be observed within DRM microdomains [30] . However, it remains unclear how FAK activation is regulated at membrane microdomains. In this study, we designed a new FRET-based FAK biosensor capable of monitoring the crucial molecular events in FAK activation: the autophosphorylation of Tyr397 and its subsequent binding to the Src SH2 domain. An improved FRET pair, ECFP and YPet, was employed to enhance the sensitivity of the FAK biosensor. This new FAK biosensor has several advantages to study the signalling hierarchy at membrane microdomains in live cells. First, the substrate peptide encompassing Tyr397 of the FAK biosensor can be specifically phosphorylated by FAK, but not by Src, a well-regarded accompanying partner of FAK [17] ( Figs 1d and 2b,c ). Hence, our new FAK biosensor enabled the crucial differentiation between the FAK and Src actions. In addition, our new FAK biosensor mimics the molecular events of FAK activation to detect its activity, but does not contain the FAK kinase domain, which may cause side effects on the downstream signalling cascades. In fact, we have shown that the PDGF-induced ERK phosphorylation, a downstream signalling event of FAK activation, was not affected by the over-expression of the FAK biosensor at various concentrations ( Supplementary Fig. S8 ), suggesting that the FAK biosensor can allow the visualization of FAK activity in live cells without perturbing the endogenous cell signalling. Finally, FRET-based FAK biosensors with Lyn- and KRas-tags are ideal to visualize the local FAK activity at dynamic membrane microdomains in live cells with high accuracy. In fact, traditional biochemical methods to isolate proteins from DRM regions may alter protein solubility during detergent treatment [6] . We observed stronger FRET responses of DRM-targeting FAK biosensor than that at non-DRM regions, on both cell adhesion and PDGF stimulations ( Figs 3 and 4 ). Indeed, DRM microdomains may provide docking platforms to concentrate FAK and facilitate its activation. This notion is in line with previous observations connecting FAK and membrane microdomains: FAK can translocate to membrane rafts on cell adhesion [31] ; The clustering of an engineered ectodomain covalently fused to a membrane-tethered FAK by antibody-coated beads can induce FAK phosphorylation [32] ; The elimination of the raft-protein caveolin blocked the FAK phosphorylation on integrin activation [33] ; The depletion of cholesterol and hence the disruption of membrane microdomains by MβCD also downregulated FAK functions [19] , and FAK regulates the localization of membrane rafts to the leading edge of a migrating cell to stabilize microtubules [20] . Furthermore, both the caveolin-containing membrane microdomains and the FAs have been shown to be highly ordered [34] , suggesting a link between raft structures and FAs. We have previously shown, with Src biosensors targeted at different membrane microdomains, that Src activation is faster and stronger at non-raft regions than at rafts [7] . Previous immunostaining results also indicate that the majority of Src is not localized at FA sites as FAK does [35] . It is hence possible that only a minor fraction of Src co-localizes with FAK at membrane microdomains, which results in the observation of a moderate Src but major FAK activation at these microdomains ( Figs 3 and 4 ) [7] . Therefore, FAK and Src can be differentially localized and regulated to result in their distinct functions. Consistently, although FAK and Src cooperate closely at FAs [17] , they have opposite effects on the development of invadopodia, which is promoted by Src, but inhibited by FAK [28] . Our results also demonstrate the differential molecular hierarchy involving FAK and Src at membrane microdomains in response to different stimulations. During adhesion process, Src activation was dependent on the enzymatic activity of FAK ( Fig. 6b ), suggesting that the FAK autophosphorylation on Tyr397, caused by its elevated kinase activity on adhesion, may recruit the SH2 domain of Src to result in Src activation. In contrast, the FAK activation on adhesion can occur in the absence of Src enzymatic activity ( Fig. 6a ), consistent with previous findings that kinase-dead Src is capable of promoting the elevation of FAK activity and rescuing the phosphorylation at Tyr 397 in SYF −/− cells [35] . Although Src kinase activity was not necessary, Src molecule was still important for the FAK activation during the adhesion process, because a complete knockout of Src family members (SYF −/− ) impaired the adhesion-mediated FAK activation ( Fig. 6a ) [36] . It is possible that the scaffolding domains of Src, for example, SH2 or SH3 domain, may regulate the FAK functions during adhesion process, either by directly causing the FAK conformational change and the exposure of its kinase domain or by recruiting other signalling molecules to modulate the FAK activity. On the other hand, Src activity was found to be required for the FAK activation, whereas the FAK activity is not essential for the Src activation on PDGF stimulation ( Fig. 5 ). Src can be activated by direct interaction between its SH2 domain and the phosphorylated PDGF receptors [37] . The activated Src kinase may then contribute to the FAK activation in various means: first, Src scaffolding domains may recruit FAK, and its enzymatic activity can directly phosphorylate the active loop in FAK, causing the full activation of FAK; or, Src may recruit other signalling molecules that can cause the open active conformation of FAK. It is interesting that FAK kinase activity has a partial effect on maintaining the PDGF-induced Src activity, although it was not required for the activation of Src ( Fig. 5b ). It is possible that the interaction between the autophosphorylated FAK Tyr397 and Src SH2 domain may be important to maintain the active conformation of Src. In summary, by monitoring the crucial molecular events in the FAK activation, we have developed a novel FRET-based FAK biosensor that allows the detection of FAK activity with high spatiotemporal resolution in live cells. The targeting of the FAK biosensor, at membrane microdomains through acylation and prenylation, can further provide powerful tools to monitor the dynamic molecular activities at subcellular compartments. Our results suggest that FAK can be activated at membrane microdomains with distinct molecular mechanisms in response to different physiological stimulations ( Fig. 7 ). Therefore, by this distinct signalling hierarchy, cells may be able to tune the different mode of responses on various physiological stimulations. 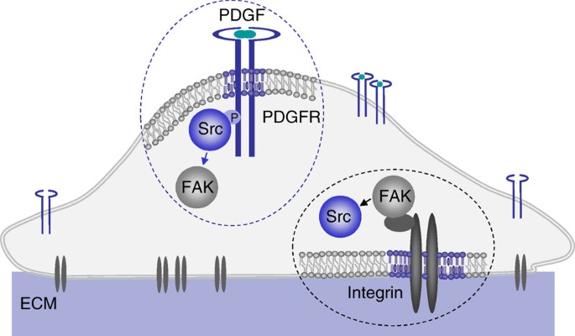Figure 7: Proposed signalling networks for the PDGF- and integrin-induced FAK signalling at membrane microdomains. The PDGF-induced FAK activation is dependent on Src. In contrast, the FAK activity and its subsequent Tyr397 phosphorylation are upstream to the Src activation in integrin-mediated adhesion processes. Figure 7: Proposed signalling networks for the PDGF- and integrin-induced FAK signalling at membrane microdomains. The PDGF-induced FAK activation is dependent on Src. In contrast, the FAK activity and its subsequent Tyr397 phosphorylation are upstream to the Src activation in integrin-mediated adhesion processes. Full size image DNA constructions The cytosolic FAK biosensor (Cyto-FAK) was constructed by fusing the SH2 domain from c-Src, a flexible linker (GSTSGSGKPGSGEGS), and a FAK substrate peptide (ETDD Y AEIIDE) between the N-terminus ECFP and the C-terminus YPet. The FAK (YF) and (RV) mutant biosensors were generated by site-specific mutations on the consensus tyrosine site (Y397F) in the substrate peptide and the critical arginine site (R175V) in the SH2 domain, using the QuikChange method (Stratagene). Lyn–FAK biosensor was constructed by adding a raft-targeting motif (M GC IKSKRKDNLNDDE) derived from Lyn kinase to the N-terminus of the Cyto-FAK biosensor [15] . KRas–FAK biosensor was constructed by adding a non-raft-targeting motif (KKKKKKSKTK C VIM) derived from KRas to the C-terminus of the Cyto-FAK biosensor [15] . The DNA encoding the FAK biosensors were subcloned with the Bam HI/ Eco RI sites in pRSetB for the protein purification from Escherichia coli , and in pcDNA3 plasmid for the expression in mammalian cells. The plasmids used in this study include the wild-type full-length FAK (FAK WT), the kinase-dead FAK with its kinase domain mutated (FAK KD), the C-terminal tail of FAK with the 1–375 amino acids truncated from the full-length FAK (FAK Δ1–375), the N-terminal tail (containing the 1–400 amino acids) of FAK (FAK NT), and the wild-type full-length of Src kinase (Src WT) [16] , [18] . Lyn-Src FRET biosensor based on ECFP/YPet was generated by adding the raft-targeting motif to the Src biosensor [14] . The GFP-tagged Akt-PH, which can bind to PIP 3 (a product of PI3K activity) and translocate to the plasma membrane on PI3K activation, was applied as an indicator to monitor PI3K activity [14] , [22] . Cell culture and reagents MEFs and FAK −/− MEF cells were maintained in DMEM supplemented with 10% fetal bovine serum (FBS), 2 mM L -glutamine, 1 unit ml −1 penicillin, 100 μg ml −1 streptomycin, and 1 mM sodium pyruvate. Cell culture reagents were purchased from GIBCO BRL. Cells were cultured in a humidified 95% air, 5% CO 2 incubator at 37 °C. Lipofectamine 2000 (Invitrogen) was used for the transfection of DNA plasmids. PDGF, fibronectin, and MβCD were purchased from Sigma. Src inhibitor PP1 was obtained from BioMol, and PI3K inhibitor LY294002 was purchased from CalBiochem. A specific FAK inhibitor PF573, 228 (PF228) [38] was obtained from Pfizer. Protein Expression The FAK biosensors were in general expressed in Escherichia coli (BL21 strain) as fusion proteins with an N-terminal 6× His tag and purified by nickel chelation chromatography [16] . Because KRas–FAK biosensor was severely cleaved when purified from BL21 cells, it was expressed in Rosetta 2 competent cells (Novagen) and purified by gel filtration on a Superdex 200 PG column (16 mm×620 mm). In brief, Rosetta 2 cells expressing KRas–FAK in the pRSETb vector were grown in LB medium (2 l) containing ampicillin (100 mg L −1 ) and chloramphenicol (25 mg L −1 ) at 37 °C with shaking at 250 r.p.m. until OD 600 measured around 1.0. Isopropyl-β- D -thiogalactopyranoside was then added to a final concentration of 0.2 mM, and the culture was incubated for another 13 h at 16 °C with shaking at 200 r.p.m.. Cells were collected by centrifugation, and re-suspended in 20 ml binding buffer (20 mM Tris·HCl, 0.5 M NaCl, 5 mM imidazole, 10% glycerol, pH 7.9) and lysed by sonication. The cell lysate was clarified by centrifugation before being applied to a 5 mL HiTrap Chelating HP column (GE Healthcare) at 4 °C. The column was washed sequentially with 50 ml binding buffer, 50 ml wash buffer 1 (20 mM Tris·HCl, 0.5 M NaCl, 50 mM imidazole, 10% glycerol, pH 7.9), and 25 ml wash buffer 2 (20 mM Tris·HCl, 0.5 M NaCl, 75 mM imidazole, 10% glycerol, pH 7.9). The column was then eluted with 25 ml elution buffer (20 mM Tris·HCl, 0.5 M NaCl, 200 mM imidazole, 10% glycerol, pH 7.9). The eluted protein was further purified by gel filtration on a Superdex 200 PG column (16 mm×620 mm) into kinase buffer (50 mM Tris·HCl, 100 mM NaCl, 10 mM MgCl 2 , pH 8). In vitro spectroscopy Fluorescence emission spectra of the purified biosensors were measured with an excitation wavelength of 430 nm by a fluorescence plate reader (TECAN, Sapphire II). The emission ratios of donor/acceptor (478 nm/526 nm) were measured before and after the addition of 1 mM ATP and recombinant FAK (1 μg ml −1 ) or Src kinase (1 μg ml −1 , Upstate) in kinase buffer (50 mM Tris·HCl, 100 mM NaCl, 10 mM MgCl 2 , 2 mM DTT, pH 8) [16] . Immunoprecipitation and immunoblotting To examine the specificity of the FAK biosensor, different FAK biosensors (wild-type and mutants) were transfected into FAK −/− MEF cells expressing the control vector, Src, FAK, or the FAK mutants. After 36–48 h of transfection, cell lysates from the various samples were subjected to immunoprecipitation with an anti-GFP antibody (Abcam) to pull down the biosensor proteins, followed by the immunoblotting with an anti-phospho-tyrosine antibody (pY20, Santa Cruz Biotechnology, 0.2 μg ml −1 ) to show the tyrosine phosphorylation level, or with an anti-GFP antibody (Santa Cruz, 0.2 μg ml −1 ) to show the expressed protein levels. The phosphorylation levels on Tyr397 and the total protein levels of the endogenous FAK were measured by a specific anti-phospho Tyr397 antibody (BD Transduction, 0.2 μg ml −1 ) and an anti-FAK antibody (Santa Cruz, 0.2 μg ml −1 ), respectively. Antibodies to detect PDGFR, ERK phosphorylation, and ERK2 were purchased from Santa Cruz Biotechnology, all with working concentration of 0.2 μg ml −1 . Sucrose density gradient fractionation MEFs expressing the Lyn- or KRas–FAK biosensor were lysed with TNE buffer (10 mM Tris, pH 7.4, 150 mM NaCl, and 5 mM EDTA) containing 2 mM PMSF, 2 mM NaF, 2 mM NaVO4, 10 nM Caluculin A, and protease inhibitor cocktail tablet. The cell lysis was centrifuged at 5,000 r.p.m. for 5 min at 4 °C. The supernatant was collected and further centrifuged at 13,000 r.p.m. for 50 min at 4 °C to obtain the membrane fractions of each group. These membrane fractions were gently reconstituted with 300 μl of lysis buffer containing 1% Triton X-100, and incubated on ice for 1 h with periodic mixing. The samples were diluted with 300 μl of 85% sucrose solution, and layered by 1.2 ml of 35% sucrose, followed by additions of 300 μl of 5% sucrose solution and 1.35 ml of TNE buffer. Ultracentrifugation was performed at 200,200 g for 18 h in a Beckman TL-100 rotor at 4 °C. After ultracentrifugation, the top 1.05 ml sample was discarded. Nine 250 μl fractions were then collected, starting from the top of the gradient, and immunoblotted with an anti-GFP antibody (Santa Cruz Biotechnology, 0.2 μg ml −1 ) to detect Lyn- and Kras-biosensors, with the Caveolin-1 antibody (sc-894, Santa Cruz, 0.2 μg ml −1 ) serving as a marker for membrane rafts regions. Image acquisition Cells were cultured in cover-glass-bottom dishes (Cell E&G) and maintained in CO 2 -independent medium containing 0.5%. FBS (Gibco BRL) at 37 °C during imaging. Images were collected by a Zeiss Axiovert microscope and MetaFluor 6.2 software (Universal Imaging) with a 420DF20 excitation filter, a 450DRLP dichroic mirror, and two emission filters controlled by a filter changer (475DF40 for ECFP and 535DF25 for YPet). The excitation filter for ECFP at 420±20 nm was selected to shift toward lower wavelength away from the peak excitation spectra of ECFP to reduce the cross-excitation of YPet and the effect of bleed-through on the FRET channel. The whole cell bodies were selected as the regions of interests to collect signals and conduct quantification. In brief, the image analysis was conducted based on the customized software written in MATLAB (version R2008a, The MathWorks). All the images were background-subtracted and smoothed using a median-filter with a window size of 3×3 pixels. The FRET images of the FAK biosensor were utilized to compute the masks of the cells using the Otsu's method where value 1 was assigned at the pixel location of cell body and 0 outside [16] . The fluorescence intensity of non-transfected cells was quantified as the background signal and subtracted from the ECFP and YPet signals of transfected cells. The pixel-by-pixel ratio images of ECFP/YPet were calculated based on the background-subtracted fluorescence intensity images of ECFP and YPet by using the MetaFluor software. These ratio images were displayed in the intensity modified display mode in which the colour and brightness of each pixel is determined by the ECFP/YPet ratio and ECFP intensity, respectively. How to cite this article: Seong, J. Detection of focal adhesion kinase activation at membrane microdomains by fluorescence resonance energy transfer. Nat. Commun. 2:406 doi: 10.1038/ncomms1414 (2011).